microTSS: accurate microRNA transcription start site identification reveals a significant number of divergent pri-miRNAs A large fraction of microRNAs (miRNAs) are derived from intergenic non-coding loci and the identification of their promoters remains ‘elusive’. Here, we present microTSS, a machine-learning algorithm that provides highly accurate, single-nucleotide resolution predictions for intergenic miRNA transcription start sites (TSSs). MicroTSS integrates high-resolution RNA-sequencing data with active transcription marks derived from chromatin immunoprecipitation and DNase-sequencing to enable the characterization of tissue-specific promoters. MicroTSS is validated with a specifically designed Drosha-null/conditional-null mouse model, generated using the conditional by inversion (COIN) methodology. Analyses of global run-on sequencing data revealed numerous pri-miRNAs in human and mouse either originating from divergent transcription at promoters of active genes or partially overlapping with annotated long non-coding RNAs. MicroTSS is readily applicable to any cell or tissue samples and constitutes the missing part towards integrating the regulation of miRNA transcription into the modelling of tissue-specific regulatory networks. MicroRNAs (miRNAs) have been a biological research hotspot since the discovery of their abundant transcription in 2001 (refs 1 , 2 , 3 ). Although significant progress has been achieved for the characterization of miRNA function, information regarding miRNA transcription regulation still remains significantly limited. Such knowledge will enable the genome-wide identification of miRNA expression regulators, including transcription factors (TFs), other non-coding RNAs (ncRNAs) and epigenetic modifiers, providing significant breakthroughs in understanding the mechanisms underlying miRNA expression in development and disease. 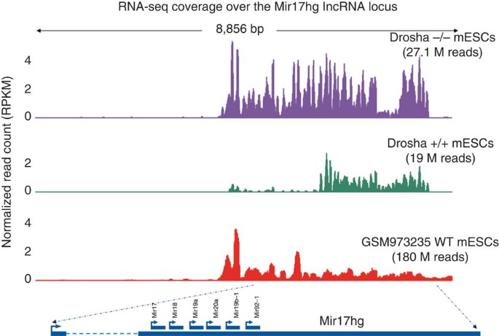Figure 1: Comparison of RNA-Seq coverage betweenDrosha−/− and wild-type mouse ESCs. The example depictsMir17hglocus transcribing a cluster of six precursor miRNAs. Purple colour represents the coverage ofDrosha−/− mouse ESCs (~27 M uniquely mapped Single End reads), while green colour is utilized forDrosha +/+ESCs (~19 M uniquely mapped Single End reads). The ‘normal-depth’Drosha +/+data set depicts the effect of Drosha processing, which is the main reason for the current lack of pri-miRNA TSS characterization. Currently annotatedMir17hgTSS is close to the start site ofDrosha +/+ Mir17hgexpression. Red colour represents the coverage of the deeply sequenced RNA-Seq data set (~250 M uniquely mapped Paired End reads) from wild-type mouse ESCs derived from the ENCODE project. This figure illustrates the ability ofDrosha−/− and deeply sequenced RNA-Seq data sets to capture the elusive pri-miRNA expression. In addition, it shows that the TSS ofMir17hgis clearly upstream from its currently annotated position. More than 45% of miRNAs ( Supplementary Table 1 ) are derived from ncRNA transcripts, while the rest are transcribed from protein-coding loci. The majority of miRNA genes are transcribed by RNA polymerase II (Pol II), generating long primary transcripts (pri-miRNAs) that are subsequently 5′ capped, spliced and polyadenylated at the 3′ end. RNase III enzyme Drosha processes pri-miRNAs into a ~60–100 nt hairpin structure termed as miRNA precursor (pre-miRNA) [4] . The rapid cleavage of pri-miRNAs by Drosha in the nucleus hinders their identification with conventional sequencing techniques. During the past few years, in silico miRNA promoter recognition methods have been elaborated as a means to address the increased difficulty of high-throughput miRNA promoter identification. Initial approaches [5] , [6] , [7] utilized DNA sequence features such as over-represented k-mers, TF weight matrices and CpG content extracted from well-annotated promoters of protein-coding genes, which were subsequently applied to identify promoters proximal to miRNA loci. These techniques provided the first indications of miRNA transcription start site (TSS) positions on a genome-wide scale. However, they exhibit high false-positive rates and require vigorous filtering and validation of the provided results. Megraw et al. [8] proposed S-Peaker, a model for ‘single-peaked TSS’ identification based solely on known TFs and their respective regions of positional enrichment. In this work, cap analysis of gene expression (CAGE) data have been utilized to derive training and test sets and categorize promoters into single-peak and multi-peak TSSs based on the width of CAGE peaks. S-Peaker provides a probabilistic score for each nucleotide in the search space upstream of miRNAs. This score reflects the nucleotide’s likelihood of being a TSS. S-Peaker supports multiple predictions per miRNA that include clusters of similarly scored nucleotides, forming peaks. Depending on the probability threshold, the width of these peaks may vary from tens up to hundreds of nucleotides. Other studies [9] , [10] , [11] utilize experimental data from active transcription marks (that is, H3K4me3, Pol II and nucleosome positioning) derived from high-throughput techniques such as chromatin immunoprecipitation sequencing (ChIP-Seq). The methodology introduced by Marson et al. [12] relies on H3K4me3 ChIP-Seq data. The algorithm considers regions enriched in H3K4me3 signals as putative promoters. An empirically derived scoring system has been deployed to score each candidate region. Positive scores were given to enriched sites if they were either the start of a known gene or an expressed sequence tag (EST) spanning the miRNA. Additional positive scores were given to enriched sites within 5 kb of the miRNA. Negative scores were assigned based on the number of intervening H3K4me3 sites and in the case where the enriched region could be assigned to a gene or EST not overlapping the miRNA. A limited amount of the algorithm’s predictions has been validated using previously characterized miRNA promoters derived from the literature. The main disadvantage of techniques utilizing active transcription marks and sequence characteristics is the underlying low-resolution and thus non-informative broad predictions. Deep sequencing data from epigenetic modifications and TF-binding motifs are indicative of broad promoter regions and are unable to support high-resolution TSS identification. For instance, the width of miRNA promoter predictions provided by the algorithm of Marson et al. [12] ranges from 0.2 to 16 kbp ( Supplementary Tables 2–4 ). miRStart [13] is a computational approach that integrates CAGE with TSS-Seq and H3K4me3 ChIP-Seq data sets. The algorithm utilizes these data to extract a signature profile around the TSS of protein-coding genes, which is subsequently considered as the basis for training a support vector machine (SVM) model. The SVM model identifies putative promoter regions upstream of mature miRNAs. miRStart filters each candidate promoter based on the distance from the corresponding miRNA and the number of overlapping ESTs or protein-coding exons. 5′ Rapid Amplification of cDNA Ends (RACE) has also been utilized to experimentally identify the promoter of liver-specific mir-122. PROmiRNA [14] is one of the latest and most advanced available algorithms. PROmiRNA utilizes CAGE data from all available tissues in FANTOM 4 database and combines them with sequence features for the characterization of miRNA promoters. It especially emphasizes in intronic miRNAs. The algorithm considers loci upstream of precursor miRNAs enriched in CAGE signals as putative promoters. Each candidate as well as randomly selected intergenic and intronic regions serve as positive and negative examples for training a probabilistic model, which additionally incorporates CpG content, conservation, TATA box affinity and mature miRNA proximity. PROmiRNA performance has been evaluated against Pol II ChIP-Seq-enriched regions and by quantifying RNA-Seq coverage between each predicted promoter and the corresponding mature miRNA. 5′ RACE has also been performed for experimentally validating the predictions of two previously uncharacterized mature miRNA promoters. miRNA TSS identification algorithms utilizing next-generation sequencing (NGS) data can be further divided into two distinct categories based on the scope of their predictions: (a) generalized algorithms and (b) experiment specific. The first group comprises algorithms integrating data derived from multiple cell lines (for example, PROmiRNA) or DNA motif analysis (for example, S-Peaker), providing multiple predictions per miRNA that correspond to different promoters, potentially active in different tissues, cell lines and conditions. These algorithms can suggest in a single run different putative miRNA TSS locations but cannot identify those active in a specific experiment (for example, cell line, treatment or tissue), since they are agnostic to its conditions. The second group (for example, microTSS, Marson et al. [12] ) utilizes NGS data from a specific experiment and provides a ‘snapshot’ of the currently active promoters in the investigated tissue or cell line. Such in silico methodologies enable experimentalists to focus only on those promoters that are active in the cell type or condition of interest and use their results as a stepping stone for building tissue-specific regulatory networks or to identify interventions. On the other hand, these methodologies require separate runs using data from different experiments, to map promoters active in different conditions. A common characteristic for existing studies in both categories is the absence of a rigid high-throughput experimental framework for validating their predictions. Well-established techniques such as 5′ RACE and reverse transcription-PCR coupled with promoter cloning are frequently utilized in the scope of miRNA promoter validation. These protocols are time consuming and low-throughput since they support single promoter validation per experiment. Most available algorithms utilized indirect means of validation (for example, existence of Poll II ChIP-Seq signals near the prediction site) and/or direct testing of selected 1-2 promoters as proof of concept. Until recently, most RNA-Seq studies provided limited sequencing depth and were not sensitive enough to capture the elusive pri-miRNA transcripts, due to increased cost and/or technical limitations. Recent improvements in deep sequencing enabled the creation of data sets comprising >200 million reads per sequenced sample. Such data are already available from extensive consortia and collaborations (for example, ENCODE consortium). The detailed analysis of such RNA-Seq data sets derived from two mouse embryonic stem cell (mESC) replicates comprising >430 million uniquely mapped reads ( Supplementary Table 5 ) revealed that pri-miRNA transcripts can be detected in data sets of high sequencing depth ( Fig. 1 ). Figure 1: Comparison of RNA-Seq coverage between Drosha −/− and wild-type mouse ESCs. 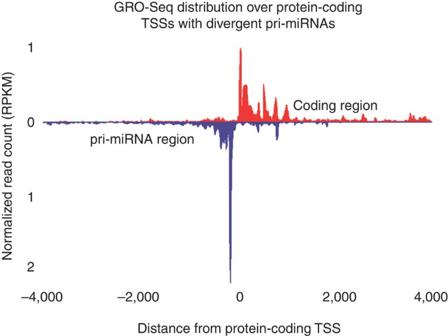Figure 5: GRO-Seq distribution around protein-coding TSSs with divergent pri-miRNAs supporting the hypothesis that divergent transcription might play an additional role in the cell by generating mature miRNAs. All identified precursor miRNAs are transcribed by the pri-miRNA region that exhibits a clear divergent transcription profile, since it fully overlaps with the GRO-Seq signal, which dissipates 2 kb upstream of coding TSSs. The example depicts Mir17hg locus transcribing a cluster of six precursor miRNAs. Purple colour represents the coverage of Drosha −/− mouse ESCs (~27 M uniquely mapped Single End reads), while green colour is utilized for Drosha +/+ ESCs (~19 M uniquely mapped Single End reads). The ‘normal-depth’ Drosha +/+ data set depicts the effect of Drosha processing, which is the main reason for the current lack of pri-miRNA TSS characterization. Currently annotated Mir17hg TSS is close to the start site of Drosha +/+ Mir17hg expression. Red colour represents the coverage of the deeply sequenced RNA-Seq data set (~250 M uniquely mapped Paired End reads) from wild-type mouse ESCs derived from the ENCODE project. This figure illustrates the ability of Drosha −/− and deeply sequenced RNA-Seq data sets to capture the elusive pri-miRNA expression. In addition, it shows that the TSS of Mir17hg is clearly upstream from its currently annotated position. Full size image We therefore hypothesized that the in silico examination of such data sets, utilizing machine-learning algorithms empowered with multiple signatures of active transcription marks, could provide accurate and high-resolution miRNA TSS identification. Importantly, extensive experimental validation of the in silico identified miRNA promoters was considered essential for the determination of the implementation’s accuracy and performance, as well as for comparison with previously elaborated methodologies. To this end, we implemented an experimental, as well as a computational framework for high-throughput miRNA TSS identification. The former consists of a Drosha - null/conditional-null ( Drosha LacZ/e4COIN ) mouse model that has been generated using the novel conditional by inversion (COIN) methodology [15] . Whole-transcriptome sequencing from mESCs derived from Drosha LacZ/e4COIN resulted to an extensive set of experimentally identified miRNA TSSs. This experimentally derived data set was kept as an independent test set, and was utilized for the thorough evaluation of the computational methods. The latter (microTSS), is an in silico approach that focuses on the identification of intergenic miRNA TSSs and relies on deeply sequenced RNA-Seq data. The algorithm integrates RNA-Seq data by creating ‘islands’ of transcription (that is, regions with increased RNA-Seq coverage) upstream of intergenic pre-miRNAs. The 5′ end of each identified expressed region is treated as a putative TSS ( Fig. 2 ). This step is the backbone of the algorithm since it provides TSS candidates with single-nucleotide resolution. A combination of three independent SVM models is subsequently utilized to score each candidate TSS and derive the final predictions. These SVM models have been trained on H3K4me3 and Pol II occupancy around protein-coding TSSs, as well as on the existence of open chromatin domains, as identified by DNase-Seq ( Fig. 3 ). 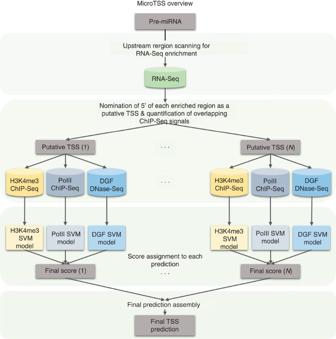MicroTSS is finally tested against TSSs identified using Drosha-null/conditional-null mESCs, as well as TSSs detected using deeply sequenced global run-on sequencing (GRO-Seq) data in human IMR90 and ES cells. Figure 2: Overview of microTSS algorithm. For each precursor, microTSS utilizes a sliding window initialized at the pre-miRNA genomic location and identifies upstream regions enriched in RNA-Seq signal. The 5′ end of each identified enriched locus is treated as a TSS candidate. The area surrounding each candidate is divided into bins of fixed/predefined size and different for each transcription marker (H3K4me3, Pol II and DNase-derived TF footprints). Each bin is assigned a score that represents the number of overlapping ChIP-Seq reads and TF footprints. Three separately trained SVM models utilize the scored bins as features and emit probabilistic estimates (one for each transcription mark), which are subsequently combined to a final score. Figure 2: Overview of microTSS algorithm. For each precursor, microTSS utilizes a sliding window initialized at the pre-miRNA genomic location and identifies upstream regions enriched in RNA-Seq signal. The 5′ end of each identified enriched locus is treated as a TSS candidate. The area surrounding each candidate is divided into bins of fixed/predefined size and different for each transcription marker (H3K4me3, Pol II and DNase-derived TF footprints). Each bin is assigned a score that represents the number of overlapping ChIP-Seq reads and TF footprints. 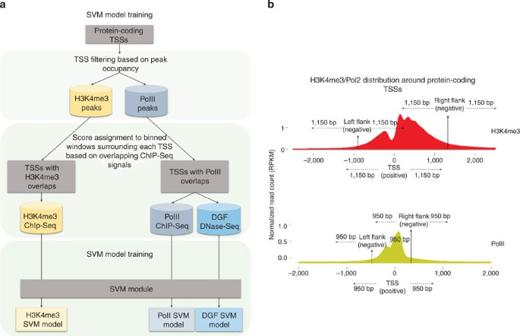Three separately trained SVM models utilize the scored bins as features and emit probabilistic estimates (one for each transcription mark), which are subsequently combined to a final score. Figure 3: SVM-training pipeline and H3K4me3/Pol II occupancy around the TSSs of protein-coding genes. (a) The initial set of protein-coding TSSs is divided into two subsets based on H3K4me3 or Pol II occupancy. The region surrounding each TSS is divided into bins and each bin is assigned a score, which is the number of overlapping ChIP-Seq reads or TF footprints. Subsequently, the scored bins are utilized as features to develop three separately trained SVMs, modelling the distribution of each transcription mark around protein-coding TSSs. (b) To train the SVM models, the annotated TSSs were selected as positive instances and the flanking regions of each active transcription mark as negatives. In addition, two randomly selected intergenic spots are selected as negatives, resulting in a 1:4 positive to negative ratio. The area (+/−1,150 and +/−950 bp for H3K4me3 and Pol II, respectively) surrounding each instance is divided in similarly scored bins of 100 nts. Both polymerase II and DGF models share the same training set, while the region (+/−2,050 bp) surrounding each DGF instance is divided in bins of 200 bps (not shown). Full size image Figure 3: SVM-training pipeline and H3K4me3/Pol II occupancy around the TSSs of protein-coding genes. ( a ) The initial set of protein-coding TSSs is divided into two subsets based on H3K4me3 or Pol II occupancy. The region surrounding each TSS is divided into bins and each bin is assigned a score, which is the number of overlapping ChIP-Seq reads or TF footprints. Subsequently, the scored bins are utilized as features to develop three separately trained SVMs, modelling the distribution of each transcription mark around protein-coding TSSs. ( b ) To train the SVM models, the annotated TSSs were selected as positive instances and the flanking regions of each active transcription mark as negatives. In addition, two randomly selected intergenic spots are selected as negatives, resulting in a 1:4 positive to negative ratio. The area (+/−1,150 and +/−950 bp for H3K4me3 and Pol II, respectively) surrounding each instance is divided in similarly scored bins of 100 nts. Both polymerase II and DGF models share the same training set, while the region (+/−2,050 bp) surrounding each DGF instance is divided in bins of 200 bps (not shown). Full size image Drosha-null / conditional-null mouse model Drosha ex4COIN/LacZ mouse model was generated to enable the identification of full-length pri-miRNA transcripts, not processed by the Drosha enzyme in the nucleus [15] . The conditional-null allele of Drosha phenocopies the null allele both in mESCs and in mice, upon conversion to the null state with Cre. Lack of Drosha enzyme expression results in an abundance of unprocessed, full-length pri-miRNA transcripts that can be readily identified ( Supplementary Fig. 1 ). Whole-transcriptome sequencing of Drosha-null mESCs resulted in the identification of 22 high-quality intergenic miRNA gene TSSs, incorporating 47 pre-miRNAs. The validated miRNA TSSs were utilized to assess the accuracy of the implemented microTSS algorithm. Comparison between Drosha-null and Drosha-wild-type Drosha-null samples exhibited significantly increased coverage of pri-miRNA regions compared with wild type (WT) ( Supplementary Table 6 ). 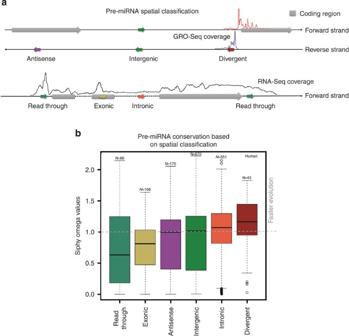Figure 6: Precursor miRNA spatial classification and conservation. (a) miRNA categories are based on their location relative to protein-coding genes. (b) Evolution rate for each spatial class as calculated by SiPhy. Divergent precursors have been found to be the least conserved group of miRNAs. Differential expression analysis was performed on the set of verified pri-miRNAs following removal of the hairpin pre-miRNA region, to identify differences in coverage of the pri-miRNA portion, which is normally cleaved within the nucleus. Fourteen (63.6%) pri-miRNA regions were significantly upregulated in Drosha-null samples, while only 2 (9.1%) were downregulated ( Supplementary Table 6 ). The majority of the experimentally derived pri-miRNA transcripts (14 out of 22) partially ( Supplementary Fig. 1 ) or fully ( Supplementary Fig. 2 ) overlap with previously annotated long ncRNA genes (lncRNAs), suggesting incomplete annotation and/or multiple functionality. Both downregulated transcripts also overlap with such loci but in their case the precursor miRNAs reside inside their introns. For instance, one of the downregulated pri-miRNA regions overlaps with Snhg4 (small nucleolar RNA host gene 4), which hosts a known snoRNA in one intron and a pre-miRNA in another. Comparison between microTSS and previous methods To construct an extensive validation set of miRNA TSSs in human, GRO-Seq data sets, derived from human IMR90 and ES cell samples published in Sigova et al. [16] and Jin et al. [17] , were analysed ( Supplementary Table 5 ). In contrast to Pol II ChIP-Seq, GRO-Seq data are strand specific. They map and quantify only transcriptionally engaged Poll II [18] . GRO-Seq density sharply peaks near the TSS in sense and antisense directions ( Fig. 4c ). A sliding window was applied on the region upstream of pre-miRNAs resulting in the identification of loci enriched in GRO-Seq signal. Regions that correlated with H3K4me3- and Pol II ChIP-Seq-derived peaks have been marked as TSSs. Precursors presenting no overlap with enriched regions have been filtered out. This pipeline resulted to the identification of TSSs for 72 pre-miRNAs in human ES and 81 pre-miRNAs in IMR90 cells. Human ESC (hESC) GRO-Seq signal around pri-miRNA TSSs is depicted in Fig. 4c . 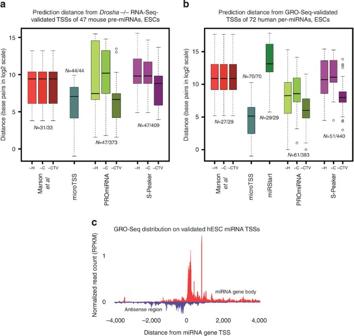These human miRNA TSSs served as two additional independent test sets. The genomic locations of the experimentally verified TSSs are presented in Supplementary Tables 7–9 . Figure 4: Comparing prediction distance from validated TSSs. PROmiRNA, S-Peaker and Marsonet al.12support multiple predictions per miRNA. The total amount of predicted TSSs is given in X/Y notation to provide a sense of precision for each algorithm. X represents the number of supported miRNAs and Y the total amount of predictions for the supported miRNAs. (a) Comparison between microTSS, S-Peaker, Marsonet al.and PROmiRNA in terms of prediction distance fromDrosha-null-validated miRNA TSSs. These are the only algorithms supporting predictions in mouse. Distance has been transformed in log2 scale. Extensions –H, –C and –CTV in PROmiRNA, S-Peaker and Marsonet al.plots represent the highest scored, the closest predictions to pre-miRNAs and closest predictions to validated TSSs, respectively. Marsonet al.supports 31 out of the 47 experimentally validated TSSs and provides 33 predictions, microTSS supports 44 TSSs by providing one prediction per miRNA while both PROmiRNA and S-Peaker support 47 TSSs and provide 373 and 409 predictions, respectively. (b) Comparing each algorithm’s prediction distance from GRO-Seq-validated TSSs of 72 precursor miRNAs in human ESCs. Marsonet al.and miRStart have been published in 2008 and 2011, respectively, thus being unable to support predictions for each of these 72 precursors. Distance has been transformed in log2 scale and differences are super-linear. Marsonet al.support 27 out of the 72 experimentally validated TSSs and provide 29 predictions, microTSS and miRStart support 70 and 29 TSSs, respectively, by providing one prediction per miRNA, while PROmiRNA and S-Peaker support 61 and 51 TSSs and provide 383 and 440 predictions, respectively. (c) Signal distribution around the GRO-Seq-validated miRNA gene transcription start site in human ESCs. Figure 4: Comparing prediction distance from validated TSSs. PROmiRNA, S-Peaker and Marson et al. [12] support multiple predictions per miRNA. The total amount of predicted TSSs is given in X/Y notation to provide a sense of precision for each algorithm. X represents the number of supported miRNAs and Y the total amount of predictions for the supported miRNAs. ( a ) Comparison between microTSS, S-Peaker, Marson et al. and PROmiRNA in terms of prediction distance from Drosha-null -validated miRNA TSSs. These are the only algorithms supporting predictions in mouse. Distance has been transformed in log2 scale. Extensions –H, –C and –CTV in PROmiRNA, S-Peaker and Marson et al. plots represent the highest scored, the closest predictions to pre-miRNAs and closest predictions to validated TSSs, respectively. Marson et al. supports 31 out of the 47 experimentally validated TSSs and provides 33 predictions, microTSS supports 44 TSSs by providing one prediction per miRNA while both PROmiRNA and S-Peaker support 47 TSSs and provide 373 and 409 predictions, respectively. ( b ) Comparing each algorithm’s prediction distance from GRO-Seq-validated TSSs of 72 precursor miRNAs in human ESCs. Marson et al. and miRStart have been published in 2008 and 2011, respectively, thus being unable to support predictions for each of these 72 precursors. Distance has been transformed in log2 scale and differences are super-linear. Marson et al. support 27 out of the 72 experimentally validated TSSs and provide 29 predictions, microTSS and miRStart support 70 and 29 TSSs, respectively, by providing one prediction per miRNA, while PROmiRNA and S-Peaker support 61 and 51 TSSs and provide 383 and 440 predictions, respectively. ( c ) Signal distribution around the GRO-Seq-validated miRNA gene transcription start site in human ESCs. Full size image By applying microTSS on deeply sequenced NGS data derived from the ENCODE consortium ( Supplementary Table 5 ) we have identified 70 intergenic miRNA gene TSSs, corresponding to 118 miRNA precursors ( Supplementary Table 10 ) in mESCs. In hESCs, we have identified 63 TSSs corresponding to 86 pre-miRNAs and in IMR90 cells 50 TSSs associated with 82 precursors ( Supplementary Tables 11 and 12 ). From the existing miRNA promoter recognition techniques, only the algorithms introduced by Marson et al. [12] , PROmiRNA [14] and S-Peaker support predictions in mouse genome. Since source codes for miRStart and Marson et al. [12] algorithms are not available, we have utilized their precompiled predictions. In addition, we took into account that these algorithms are based on outdated miRBase versions, comprising fewer miRNAs than miRBase v20 (ref. 19 ), which is utilized by microTSS, PROmiRNA and S-Peaker. Therefore, the prediction set of these algorithms has been reduced to the annotation utilized for their implementation. Some of the algorithms that we have identified offer multiple TSS predictions per miRNA, while others offer a single prediction. To perform a robust comparison and account for the fundamental differences between the algorithms in both categories we established two distinct evaluation pipelines. In the first approach, we have selected one prediction per miRNA for each method. For the algorithms in the first category, this corresponds to the standard set of supported predictions. On the other hand, for the methods in the second category, three distinct subsets of predictions have been created. The first (denoted with the extension –H) comprises the highest scored TSSs in the region upstream of miRNAs, while the second includes the closest predictions to each precursor (denoted with the extension –C). The last subset contains the closest predictions to the experimentally verified TSS (denoted with the extension –CTV). It should be noted that the last set (–CTV) requires a priori knowledge of the true TSS to be defined and can be applied from the user if all predictions per miRNA are taken into account. The distance of all predictions relative to the corresponding validated TSSs has been calculated and the number of all predictions is also noted ( Fig. 4a,b ; Supplementary Figs 3–6 ), including descriptive and inferential statistics ( Supplementary Tables 13–15 ). It can be observed that microTSS performs significantly better than all the other programs of the same category exhibiting median distance, between the predicted and validated TSS, smaller than 35 nts in human and 130 nts in mouse. MicroTSS outperforms the –C and –H sets of the programs in the second category (where one prediction per miRNA has been selected) and is comparable to the –CTV set, where the closest predictions to the validated TSSs (out of several predictions for each miRNA) have been used. In the second evaluation pipeline, the predictions provided by the algorithms have been utilized to measure their sensitivity and precision. To this end, we have applied a threshold of 1,000 bp on the prediction distance from validated TSSs. Predictions located closer than 1 kbp from the validated TSS are considered true positives (TPs) and the rest are treated as false positives (FPs). Precision has been calculated as the number of TPs divided by the number of total predictions (TPs+FPs). Sensitivity is defined as the number of TPs divided by the number of positives (supported miRNAs from the validation set). Marson et al. [12] achieves 54 and 64.5% in mESCs, 15.2 and 40.7% in hESCs, 18.5 and 29.4% in IMR90 sensitivity and precision, respectively. miRStart on the other hand, achieves 5.5%/4.9% and 13.7%/10.8% sensitivity and precision in hES/IMR90 cells. MicroTSS significantly outperforms the algorithms of the same category by exhibiting 93.6 and 100% in mESCs, 94.4 and 97.1% in hESCs, 91.3 and 91.3% in IMR90 sensitivity and precision, respectively. The algorithms of the second category that provide multiple TSS predictions per miRNA, possibly active in different cell types/tissues (that is, PROmiRNA and S-Peaker), have been excluded from this evaluation pipeline since the evaluation sets consist only from promoters specifically active in the investigated cell lines. These results depict the fundamental differences between the methodologies of the two categories. Algorithms such as PROmiRNA and S-Peaker provide high-quality predictions close to the validated TSS (–CTV results) but are often lost within numerous predictions, since in most cases they are not highly scored. This results in an increased FP rate due to the high number of predictions per miRNA decreasing prediction precision. On the other hand, microTSS addresses this issue by utilizing expression data from the investigated cell line or tissue, providing single predictions per miRNA close to the validated TSS and provides a ‘snapshot’ of the currently active promoters. The unique combination of high precision and sensitivity provided by microTSS enables the study of miRNA regulation and their complete integration in cell line-/tissue-specific regulatory networks. MicroTSS performance on variable RNA-Seq depth and coverage Sequencing depth and the algorithm’s sliding-window threshold of RNA-Seq coverage are key parameters in microTSS performance. To assess their effects on the algorithm’s outcome, we have performed two distinct tests. In the first test ( Supplementary Fig. 7a ), random subsampling has been applied on the WT mESC RNA-Seq data (GSM973235) resulting in four subsets of 20, 40, 60 and 80% of the initial data set’s depth (2 × 125 M uniquely mapped, strand-specific, paired-end reads). The performance of microTSS on each subset has been evaluated using the set of Drosha −/−-validated TSSs. The analysis suggests that even at lower sequencing depths (for example, 2 × 25 M uniquely mapped reads), microTSS is able to accurately identify TSSs corresponding to the most abundant pri-miRNAs and expressed precursors, that is, miRNA transcripts with low degradation rate. Gradual increments in the sequencing depth enable microTSS to capture pri-miRNAs and precursors of lower abundance and expression rate, respectively. In the second test ( Supplementary Fig. 7b ), microTSS has been applied on the same WT mESCs RNA-Seq data set (GSM973235) by utilizing four different thresholds for the RNA-Seq coverage. The threshold of five reads, which is the default, is able to identify TSSs of pri-miRNAs with a high degradation rate without compromising the prediction accuracy. The algorithm is less sensitive, at the same levels of precision, as the threshold increases. Polycistronic pri-miRNAs and coverage of annotated lncRNAs The analysis of microTSS predictions revealed that 37.1% of TSSs in mESCs (26 out of 70), 19% in human ESCs (12 out of 63) and 30% (15 out of 50) IMR90 cells are associated with multiple pre-miRNAs. miRNAs (40.6%) in hESCs (35 out of 86), 57.3% in IMR90 cells (47 out of 82) and 62% in mECSs (74 out of 118) are derived from polycistronic miRNA gene clusters. Moreover, 28% of TSSs in mESCs (20 out of 70), 25.3% in hESCs (16 out of 63) and 44% in IMR90 (22 out of 50) correspond to pri-miRNAs that partially or fully overlap with already annotated lncRNA genes. For example, our findings regarding mouse pri-mir-675 are in agreement with previous studies [20] , [21] showing that it fully overlaps with H19 lncRNA gene, which has been found to control several genes within the imprinted gene network. H19 recruits MBD1 and forms a lncRNA:protein complex that interacts with histone lysine methyltransferases and represses its target genes [21] . A recent study has also revealed that H19 hosts both canonical and non-canonical binding sites for the let-7 family, thus acting as a molecular sponge [20] . Another example of incomplete annotation is Mir17hg , which has been classified as a small RNA host transcript [22] . The analysis of microTSS predictions shows that Mir17hg is a polycistronic miRNA gene cluster, hosting 6 precursors (mir-20a, mir-17, mir-19b-1, mir-18a, mir-92a-1 and mir19a) whose identified TSS is located several hundred base pairs upstream of the current annotation. The analysis of small-RNA-Seq data in mESCs ( Supplementary Table 16 ) revealed different patterns of pre-miRNA expression in polycistronic miRNA genes. There are cases where all members of the same cluster share similar expression levels. Mir-365-1 and mir-193b are transcribed from the same pri-miRNA exhibiting very low RPKM values. In other cases, co-clustered miRNAs present significantly different expression levels. D7ertd143e polycistronic miRNA locus hosts mir-292, mir-291a, mir-295, mir-293 and mir-294 located in the top 64 expressed pre-miRNAs in mESCs, while the remaining two precursors of the cluster, mir-290a and mir-291b, exhibit significantly lower expression levels. These results are in agreement with previous studies suggesting that there are post-transcriptional mechanisms responsible for blocking individual members of polycistronic miRNA genes from the maturation process. In a recent study [23] , adenosine deaminases acting on RNAs ( ADARs ) were shown to alter the structural conformation of let-7 polycistronic pri-miRNA transcript, resulting in limited Drosha processing for individual members of the cluster and enhanced processing for others. Divergent antisense pri-miRNAs identified with GRO-Seq Several recent studies have shown that the majority of mammalian promoters initiate transcription on both sense and antisense directions, a phenomenon known as divergent transcription [24] , [25] . Divergent transcription generates upstream antisense RNAs near the 5′ end of genes that are typically short (50–2,000 nucleotides) and in many cases unstable [26] . These results suggest that the common phenomenon of divergent transcription of active promoters may help promoter regions to maintain a state poised for subsequent regulation and has been proposed as a model for new gene formation [26] . In mouse and human ESCs, divergent transcription from promoter and enhancer regions of protein-coding genes is the major source of intergenic transcription [26] . The analysis of microTSS predictions based on their distance from protein-coding genes revealed a significant number of precursors residing very close to coding loci. We subsequently performed spatial classification of all pre-miRNAs in miRBase identifying 13 (1.1%) putative divergent miRNAs in mouse and 43 (2.3%) in human, based on the distance to their corresponding protein-coding gene ( Supplementary Table 1 ). To validate that these pri-miRNAs are indeed transcribed divergently upstream from active protein-coding gene promoters, we analysed mouse and human ESC GRO-Seq data. Eleven out of 13 (84.6%) mouse divergent miRNAs TSSs ( Supplementary Table 17 ) and 26 out of 43 (60.4%) human ( Supplementary Table 18 ), exhibit divergent GRO-Seq signals 2–3 kb upstream of the closest protein-coding gene, fully overlapping with expressed regions of these miRNA precursors ( Fig. 5a ). Six out of 11 (54.5%) mouse and 11 out of 26 (42.3%) human GRO-Seq-verified divergent pri-miRNAs have also been identified using microTSS algorithm and deep ESC RNA-Seq data, further supporting our initial hypothesis. miRNA precursors from such loci are significantly less conserved, consistent with the recently proposed model of new gene formation [26] . Relevant graphs and descriptive as well as inferential statistics are presented in Fig. 6 ; Supplementary Table 19 . Figure 5: GRO-Seq distribution around protein-coding TSSs with divergent pri-miRNAs supporting the hypothesis that divergent transcription might play an additional role in the cell by generating mature miRNAs. All identified precursor miRNAs are transcribed by the pri-miRNA region that exhibits a clear divergent transcription profile, since it fully overlaps with the GRO-Seq signal, which dissipates 2 kb upstream of coding TSSs. Full size image Figure 6: Precursor miRNA spatial classification and conservation. ( a ) miRNA categories are based on their location relative to protein-coding genes. ( b ) Evolution rate for each spatial class as calculated by SiPhy. Divergent precursors have been found to be the least conserved group of miRNAs. Full size image The analysis of precursor miRNAs in mESCs ( Supplementary Table 16 ) revealed that out of the 11 GRO-Seq-validated divergent pre-miRNAs, only mir-320 was highly expressed in the small-RNA-Seq sample. Mir-1934, mir219c and mir-345 have been found to exhibit very low expression levels, and the rest have not been detected at all. These four precursors correspond to only 8 out of 24 mature divergent miRNA candidates. Mir-320 and mir-345 are highly conserved and divergently transcribed from Polr3d and Slc25a29 , respectively ( Supplementary Tables 17 and 18 ). Out of the expressed divergent precursors in this cell line, only these two miRNAs were identified to interact with coding genes in TarBase v6 (ref. 27 ), an extensive database of experimentally supported miRNA:gene interactions. In fact, mir-320 targets the same gene ( Hspb6 ), among many others, in both species as well as its adjacent gene ( Polr3d ) in human. Mir-345 has been found in the same database to interact only with three genes in human. At the same time the in silico analysis of divergently transcribed miRNAs with microT-CDS [28] provide a significant number of targets for all miRNAs. The small-RNA-Seq analysis further revealed that out of the 99 mature miRNAs located in expressed intergenic transcripts, close to 20% (20 mature miRNAs) reside in divergently expressed loci, while in the small-RNA-Seq data set, they correspond to a ~2% fraction (8 out of 411 expressed mature intergenic miRNAs). This is an indication that these divergently transcribed miRNAs are more often repressed on a later stage of miRNA biogenesis, exhibiting a significantly smaller transcription versus expression ratio, as identified with GRO-Seq and small-RNA-Seq, respectively ( P <10 −12 ). We have identified more miRNAs expressed using the small-RNA-Seq data set than trancribed, as identified by the GRO-Seq data. Although both data sets have comparable numbers of reads, in our opinion the underlying cause is small-RNA-Seq’s strict size fractionation, which restricts the available sequencing depth to miRNA-specific RNA lengths. Knockout/conditional knockout models of genes central to the miRNA biogenesis pathway, such as Dgcr8 or Dicer have been previously utilized to assess and quantify alterations in miRNA expression and function between wild-type samples and knockouts, or to identify miRNAs generated by non-canonical pathways [29] , [30] . To our knowledge, this is the first available study implementing a Drosha conditional allele animal model for the study of unprocessed pri-miRNA transcripts. This mouse model was generated using COIN technology [15] , which is an exceptionally robust and universal method that can be applied to all genes, regardless of their size and structure, overcoming any limitations of previous relevant techniques. The utilized mouse enabled for the first time a high-throughput pri-miRNA transcript identification using conventional RNA-sequencing. Recent advances in the field of NGS resulted in a concurrent cost reduction and quality increase of derived data. As demonstrated in this study, detection of intergenic pri-miRNAs is now achievable with the use of deeply sequenced transcriptomic RNA-Seq, ChIP-Seq and DNase-Seq experiments. Such data can be analysed using microTSS, to provide accurate and high-resolution miRNA TSS predictions. The novelty of the algorithm resides in its ability to integrate tissue-specific deeply sequenced RNA-Seq data, resulting in single-nucleotide TSS predictions. It is able to detect TSSs currently active in cell lines or conditions of interest. Highly precise predictions will enable comparison between states and integration of ncRNA regulators in tissue-specific networks. The implemented experimental and computational methods are readily applicable to other cell lines or organisms and can become essential tools for high-throughput miRNA TSS identification. These methodologies can be utilized separately or combined, depending on the study setting, availability of data sets and genome annotation of the examined organism. Such high-quality results constitute an invaluable resource towards the characterization of the elements regulating miRNA expression. The analysis of microTSS predictions in mES, hES and IMR90 cells showed that a significant number of pri-miRNAs overlap partially or completely with previously annotated lncRNAs. These findings suggest incomplete annotation of certain non-coding loci and/or multiple functionality. This hypothesis is supported by previous studies showing that many lncRNAs are retained in the nucleus acting as pri-miRNAs or they are exported to the cytoplasm and serve as post-transcriptional regulators of gene expression, playing distinct roles that can be tissue specific [20] , [21] . MicroTSS is a resource able to facilitate the annotation of pri-miRNAs and non-coding transcripts in general, as well as to support targeted functional studies of lncRNAs. MicroTSS results have revealed novel dicistronic and polycistronic miRNA transcripts. The analysis of small-RNA-Seq data in mESCs has additionally depicted variable expression levels between co-clustered precursors. There are cases where specific miRNAs exhibit no or low expression as compared with other members of the same cluster. Such observations have also been reported in previous studies [23] , suggesting post-transcriptional mechanisms able to block the maturation process of individual members derived from polycistronic miRNA genes.The analysis of GRO-Seq data unveiled a significant number of divergent pri-miRNAs upstream of protein-coding gene promoters. The significantly smaller degree of conservation in these precursor sequences directly supports the proposed hypothesis [26] that divergent transcription is a model of new gene formation. The analysis of long- and small-RNA-Seq data in mouse indicates that the maturation process of miRNAs located in divergent transcripts is repressed more often than expected on a later stage. Although the small RNA data set is deeply sequenced, we cannot exclude the possibility that these miRNAs are expressed below its detection limit. However, even in this case there is a strong indication that their rate of maturation is either blocked or actively regulated. It can also be connected to the aberrant divergent transcription observed in ES cells, serving as a means of cell protection from redundant miRNA transcription. Only a few of the miRNAs located in divergent transcripts had experimentally validated targets, but all were predicted to have a significant number of in silico identified interactions. It could be possible that processing of divergent miRNA transcripts is more difficult to be regulated since it is not independent from the transcription of adjacent protein-coding genes. A recently discovered mechanism [23] enables cells to distinguish miRNAs located in the same polycistronic transcript by blocking others and preferentially allowing only their maturation. The existence of this additional layer of post-transcriptional miRNA biogenesis regulation might be the only way to enable the preferential tissue- or cell line-specific expression/repression of divergent miRNAs (and other monocistronic pri-miRNAs). Future experiments in multiple tissues would provide valuable information towards the evaluation of this hypothesis. Previous studies [12] have attempted to incorporate miRNA expression into the framework of gene regulatory networks. An additional layer of controlling gene expression has been proposed that involves miRNAs by serving as positive and negative regulators by fine-tuning the effects of TFs on their target genes in coherent and incoherent feed-forward networks. The discovery of such mechanisms is an endeavour that requires accurate genome-wide characterization of miRNA TSSs specific to each case study or experimental setup. MicroTSS is the only available algorithm that provides tissue-specific, highly accurate intergenic miRNA TSS predictions. This can be achieved by utilizing experimental data from any cell condition, cell type and tissue enabling microTSS to be an invaluable resource towards the accurate identification of miRNA regulatory elements (for example, TFs, lncRNAs and epigenetic modifications). The identification of differences in miRNA expression regulation between pathological and physiological conditions, cell types and species, could inaugurate a new era for the elucidation of miRNA expression and redefine their role into the wider context of biological pathways. Drosha-null and Drosha-wild-type data generation Drosha-null mESCs were generated by treating Drosha ex4COIN/LacZ ; Gt(ROSA)26Sor CreERt2/+ cells with Tamoxifen (500 ng ml −1 ) to activate the CreERt2 recombinase, and clones with inverted COIN module were identified, one of which (LD12) was used in this study. LD12 exhibits abrogation of Drosha expression and absence of a mature microRNA miR-293, and concomitant accumulation of its precursor pri-miR-293, indicating lack of Drosha functionality [15] . Mouse ES cells of WT or Drosha-null genotype were cultured on gelatinized plates free of feeder cells. Total RNA was extracted using the miRNeasy Mini Kit (Qiagen). Two μg of total RNA was converted to poly(A)+ RNA using oligo-dT-coated magnetic beads (Invitrogen). Poly(A)+ RNA was converted to strand-specific Illumina sequencing libraries with 8-bp barcodes using the Epicenter ScriptSeq V1 RNA-Seq library preparation kit (Epicenter, Illumina Inc, USA). RNA-Seq libraries were hybridized to a single-end flow cell and individual fragments were clonally amplified by bridge amplification on the Illumina cBot. Upon completion of clustering, the flow cell was loaded on the HiSeq 2000 (Illumina Inc) and sequenced using Illumina’s SBS chemistry. Samples were run for 33-bp sequencing reads as well as 9-bp index reads. Base call (.bcl) files for each cycle of sequencing were generated by Illumina Real Time Analysis software and de-multiplexed to FASTQ files, which were used for analysis in this study. RNA-Seq and GRO-Seq analysis Apart from the generated Drosha −/− and +/+ RNA-Seq data sets, mESC RNA-Seq data have been derived from the ENCODE consortium repository (GEO accessions GSE49847 and GSM758574 ). GRO-Seq data were obtained from the studies of Min et al. [31] (GEO accession GSE27037 ), Sigova et al. [16] (GEO accession GSM1006728 ) and Jin et al. [17] (GEO accession GSM1055806 ). Quality control has been performed using FastQC ( www.bioinformatics.babraham.ac.uk/projects/fastqc ). Contaminants were detected and removed utilizing a combination of an in-house developed algorithm and already available tools such as minion [32] and trimgalore ( www.bioinformatics.babraham.ac.uk/projects/trim_galore ). Following pre-processing, GSNAP spliced aligner [33] was utilized to map the reads against the reference genomes (GRCm38/mm10 and GRCh37/hg19 genome assemblies). GSNAP has been appropriately parameterized to detect novel and known splice junctions. The analysis resulted in ~849 M uniquely mapped Paired End reads (WT RNA-Seq), ~27 M uniquely mapped Single End reads ( Drosha-null mESCs RNA-Seq) and ~288 M uniquely mapped Single End reads (wild-type GRO-Seq). GRO-Seq data were aligned against the genome using Bowtie v1 (ref. 34 ). Reads aligned to >1 genomic location have been discarded from subsequent analyses ( Supplementary Table 5 ). Differential expression analysis was performed using EDGER [35] . Small-RNA-Seq analysis ESC small-RNA-Seq data were derived from the study of Chang et al. [36] (GSM886478). Following pre-processing, adapter-trimmed reads were aligned against known human mature miRNA sequences (miRBase v20 (ref. 19 )) using Bowtie v1 ref. 34 . Unaligned reads were subsequently mapped against known pre-miRNAs (miRBase v20 (ref. 19 )). Reads mapped on pre-miRNAs not clearly overlapping a mature miRNA sequence were discarded. Alignments on identical mature miRNAs deriving from distinct pre-miRNAs were collapsed. Identification of the miRNA expression was finally estimated on mature miRNA level by combining both alignment results. ChIP-Seq and DNase-Seq analysis ESC raw H3K4me3 and Pol II ChIP-Seq data have been derived from the published collection of Shen et al. [37] , Derrien et al. [38] and Jin et al. [17] . Quality control and contaminant removal was performed using the same tools and techniques as for RNA-Seq and GRO-Seq data. Bowtie v1 (ref. 34 ) has been utilized to align the reads to the reference genome (GRCm38/mm10 and GRCh37/hg19 genome assemblies). The analysis resulted in ~42 and ~47 M uniquely mapped H3K4me3 and Pol II reads, respectively. SICER [39] and Macs2 (ref. 40 ) have been used to identify enriched regions in H3K4me3 and Pol II signals. Digital genomic footprinting (DGF) data produced by DNase-Seq have been derived from the ENCODE consortium repository (GEO accessions GSE40869 , GSE32970 and GSM1008586 ) and the migration from mm9 to mm10 has been accomplished using liftover tool provided by University of California Santa Cruz ( Supplementary Table 5 ). The integration of these data sets has facilitated the training and optimization processes of the SVM models. Description of the algorithm MicroTSS is composed of two distinct modules ( Fig. 2 ). Initially, the algorithm identifies regions enriched with RNA-Seq reads upstream of intergenic pre-miRNAs. This is accomplished by utilizing a sliding window initialized at the pre-miRNA genomic location, covering a user-defined distance. Each window is assigned a score that represents the number of overlapping RNA-Seq reads. The applied window size, sliding step and score threshold are also parameterized. We suggest 30 nts as default length for the sliding window and the relevant score threshold at 5 overlapping RNA-Seq reads ( Supplementary Fig. 7b ), regardless of sequencing depth. These are microTSS recommended default values that result in maximum sensitivity without compromising the algorithm’s accuracy. The default sliding-window step has been set to 5 nts, which provides fast execution and increased accuracy. MicroTSS filters out windows according to the threshold score and merges the remaining ones based on a user-defined distance, enabling the identification of genomic loci enriched in RNA-Seq reads. Assessing the performance of the algorithm for a wide range of this parameter values, we observed that a robust selection, in terms of sensitivity and precision, is 200 nts. The length of the scanning region upstream of each pre-miRNA has been set to 400 kbp. This value has been selected based on previous studies that have identified TSSs located >100 kbp away from their corresponding precursors and in some cases even 150 kbp. All settings can be altered by microTSS users, to cater different experimental aims and study designs. The 5′ ends of the identified RNA-Seq-enriched loci serve as putative TSSs. Subsequently, microTSS combines three SVM models to score each putative TSS and to filter out FPs. The SVM models have been trained on H3K4me3 and Pol II ChIP-Seq, as well as DGF TF-binding occupancy ( Supplementary Table 20 ) on a set of annotated protein-coding genes ( Fig. 3 ). Each candidate TSS position is assigned three different windows of varying size, depending on the corresponding SVM model. The H3K4me3 window length is +/−1,150 bp around the candidate TSS, while the Pol II and DGF are +/−950 bp and +/−2,050 bp, respectively. The H3K4me3 and Pol II windows are divided in bins of 100 nts, while DGF are divided in bins of 200 nts. Each bin is assigned a specific score, which is the number of overlapping ChIP-Seq reads or TF footprints. The scores for all bins are subsequently forwarded to the SVM models as features, which in turn estimate the probability for the candidate position to actually include a bona fide TSS. The final score of each candidate TSS is the sum of the three probabilities. Cases exhibiting a final score below a threshold are filtered out. From the remaining candidates, microTSS reports the one corresponding to the highest final score. The default threshold for the final score is set to 1.5. Selection of a lower threshold would increase sensitivity in the risk of incorporating ambiguous predictions. SVM model training The promoters of miRNA genes have been shown to present similar characteristics with protein-coding genes, since their transcription is regulated by Pol II. H3K4me3, Pol II and TFs are considered key elements in the initiation of gene transcription. H3K4me3 has been found to occupy the promoters of actively transcribed genes or genes poised for transcription. TFs are required for recruiting the transcription machinery, which is driven by Pol II. Due to the observed underlying hierarchy in promoter occupancy, in many cases TSSs of protein-coding genes have been found to correlate only with H3K4me3 peaks, others have been shown to be occupied by H3K4me3 and TFs, while the majority is controlled by all three transcription marks. To properly capture the information residing in each proposed active transcription mark, three distinct SMV models have been trained on a set of annotated protein-coding TSSs derived from Ensembl v74 (ref. 41 ), utilizing ChIP-Seq data against H3K4me3 and Pol II as well as DGF TF-binding sites ( Fig. 3 ). The training procedure has been accomplished using libsvm v3.0 (ref. 42 ), which provides probability estimations instead of performing binary classification. Radial basis function has been chosen over the linear kernel since it performed better in cross-validations. ChIP-Seq signals corresponding to TSSs of multiple genes with an in-between distance smaller than 10 kbp have been filtered out. The finalized set of protein-coding genes comprises 10,929 entries. This group of genes has been subsequently divided into two sets with a ratio of 4 to 1: 8,740 TSSs were utilized for training and 2,189 for testing the SVM models. SICER [39] and Macs2 (ref. 40 ) have been applied to identify genomic locations (peaks) enriched in H3K4me3 and Pol II, respectively, enabling the development of a robust predictive model. Peaks exhibiting a false discovery rate (FDR) higher than 0.05 have been filtered out. Out of the 8,740 protein-coding genes in the training set, 4,504 have been found to overlap with H3K4me3 peaks and 1,623 with Pol II peaks ( Supplementary Table 20 ). To train each model, the centre of each peak served as a positive instance while the leftmost and rightmost positions were treated as negatives. In addition to the flanking positions of the peak, two randomly selected intergenic spots are selected as negatives, resulting in a 1:4 positive to negative ratio ( Fig. 3 ). To develop a robust DGF model, its training set should consist of promoters with fully recruited TF machineries. This could only be the case for promoters occupied by Pol II. Thus, the set of protein-coding genes utilized for training the Pol II model has also served as training set for the DGF SVM model. Ten-fold cross-validation has been performed on the training data to estimate the performance of each model, achieving 98% accuracy for the DGF model, 98% for the Pol II model and 99% for the H3K4me3 model ( Supplementary Table 20 ). The protein-coding test set was utilized to evaluate the performance of the final combined model, as well as to estimate its generalization ability and to avoid overfitting. Even by applying a loose threshold on the final score of each prediction (as explained in the previous section) the algorithm can predict TSSs of the unknown test genes with 99.5% accuracy, 98.2% precision, 99.5% specificity and 99.7% sensitivity ( Supplementary Table 20 ). MicroTSS was initially developed to combine H3K4me3, Pol II and TF occupancy within a single model. However, this approach resulted in H3K4me3 consistently overshadowing/masking the other marks’ properties. H3K4me3 consistently occupies TSSs, but its binding region tends to be very wide. Pol II and DGFs on the other hand, occupy fewer TSSs than H3K4me3 but in a significantly narrower region. Supplementary Fig. 8 demonstrates the size of the binding region of each transcription mark, suggesting that all three features are informative and equally important. The score of each model acts as additive value/evidence strengthening the likelihood of each candidate TSS and removing the majority of FPs. The distribution of the score provided by each individual model remains unaffected by the expression level and is similar for both protein-coding and miRNA genes. Precursor miRNA spatial classification and conservation Human and mouse pre-miRNAs have been divided into six categories depending on their genomic location relative to protein-coding genes ( Fig. 6a ). Precursors residing inside protein-coding exons/introns have been classified as ‘exonic’/‘intronic’. miRNAs located in the opposite strand of protein-coding loci were classified as antisense. Pre-miRNAs located in the immediate (<4,000 bp) upstream/downstream sense region of protein-coding genes have been labelled as read-through. RNA-Seq signal profile at these loci suggests common transcription regulation for both coding and non-coding genes. On the other hand, miRNAs located in the upstream antisense region (<2,000 bp) of coding loci were classified as divergent. The remaining precursors were characterized as intergenic ( Supplementary Table 1 ). To identify the evolutionary rate of each category, multiple alignment files between 21 mammals in MAF format have been downloaded from the University of California Santa Cruz repository. SiPhy [43] has been utilized to calculate the local rate of substitutions compared with a neutral phylogenetic tree model, which is depicted in the estimated omega values. Higher omega scores are associated with less-conserved regions and precursors surpassing the cutoff value 1.0, as determined by SiPhy, are considered rapidly evolving sequences. Due to the limited amount of identified divergent miRNAs in mouse, statistical analysis on the conservation results has been performed only for human precursors. How to cite this article : Georgakilas, G. et al. microTSS: accurate microRNA transcription start site identification reveals a significant number of divergent pri-miRNAs. Nat. Commun. 5:5700 doi: 10.1038/ncomms6700 (2014). Accession codes. Raw and processed RNA-seq data for Drosha +/+ and Drosha −/− mESCs samples have been deposited in Gene Expression Omnibus (GEO) under accession code GSE55735 . Source code availability. The source code for microTSS is available at www.microrna.gr/microTSS .